Spin coupling and relaxation inside molecule–metal contacts Advances in molecular electronics depend on the ability to control the charge and spin of single molecules at the interface with a metal. Here we show that bonding of metal–organic complexes to a metallic substrate induces the formation of coupled metal–ligand spin states, increasing the spin degeneracy of the molecules and opening multiple spin relaxation channels. Scanning tunnelling spectroscopy reveals the sign and magnitude of intramolecular exchange coupling as well as the orbital character of the spin-polarized molecular states. We observe coexisting Kondo, spin, and vibrational inelastic channels in a single molecule, which lead to pronounced intramolecular variations of the conductance and spin dynamics. The spin degeneracy of the molecules can be controlled by artificially fabricating molecular clusters of different size and shape. By comparing data for vibronic and spin-exchange excitations, we provide a positive test of the universal scaling properties of inelastic Kondo processes having different physical origin. Metal–organic molecules provide a rich variety of charge and spin states that can be used to tailor the conductance of single-molecule electronic devices [1] , [2] , [3] . Strong nonlinear current-voltage effects, such as negative differential resistance, Coulomb-blockade, Kondo and vibrational resonances have been observed in three-terminal measurements of molecules trapped between metal electrodes [1] , [2] , [3] , [4] , [5] , stimulating proposals for integrating metal–organic complexes into information processing architectures [6] . A key step in this quest is to reveal how the molecular spin couples to electrons inside and outside a molecule, providing different pathways for spin excitation and relaxation. This cannot be fully accomplished in 'blind' molecular junction experiments, as the molecule environment is often hardly reproducible and poorly characterized [7] , [8] . Here we use spectroscopic imaging by scanning tunnelling microscopy (STM) to elucidate the origin, intramolecular density, and coupling of the spin magnetic moment in metal–phthalocyanine molecules adsorbed on the Ag(100) surface. We show how bonding to a metal electrode modifies the electronic energy spectrum and spin degeneracy of both magnetic and nonmagnetic molecular adsorbates, opening different spin coupling and relaxation channels with distinctive spatial localization and decay rates. The emerging picture illustrates how the atomic configuration of the contact in a molecular junction will determine not only the hybridization of molecule–metal states, and hence the elastic conductance, but also select the type of inelastic excitations that dominate spin decoherence al low energies. Pristine spin moment and adsorption of CuPc and NiPc on Ag(100) Metal–phthalocyanine are representative of a broad class of planar metal–organic complexes with several applications in organic electronics [9] . Our study focuses on CuPc and NiPc, owing to their simple magnetic properties and well-defined ionic spin moment. Before adsorption, CuPc is paramagnetic with spin S=1/2 owing to an unpaired electron residing in the d x 2- y 2 (b 1 g ) metal orbital, whereas NiPc is diamagnetic with S=0 (ref. 10 ). 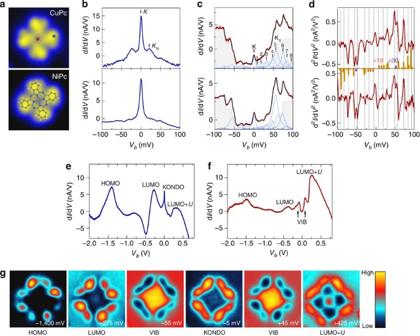Figure 1: Structure and electronic properties of paramagnetic CuPc and diamagnetic NiPc adsorbed on Ag(100). (a) STM image of single CuPc (top,I=72 pA,Vb=−5 mV) and NiPc (bottom,I=100 pA,Vb=−3 mV), image size 2.5 nm×2.5 nm. The diagram superposed to NiPc indicates the position of the metal (orange), C (grey), N (blue), and H (white) atoms. (b) dI/dVspectra of CuPc (top) and NiPc (bottom) aroundEFmeasured on benzene (blue dot) and (c) on Cu and Ni ions (red dot) (setpoint:I=2 nA/1.1 nA,Vb=−100 mV for CuPc/NiPc). Labels denote Kondo resonances of different nature: zero-bias (K), triplet–singlet (Kts), and vibrational (Kv). Black solid lines incare fits to the data using the sum of Lorentzian (blue) and step functions (shaded). (d) d2I/dV2spectra of CuPc (top) and NiPc (bottom) measured on Cu and Ni ions. The dashed lines indicate the energy of the step excitations inc, which correspond to the amplitude of the Raman-active vibrational modes of gas-phase CuPc (bars)21. (e) Extended dI/dVspectra of CuPc on benzene and (f) Cu sites (setpoint:I=3 nA,Vb=−2 V). (g) dI/dVmaps of the molecular orbitals and inelastic vibrational signal shown ineandftogether with the d2I/dV2map of the Kondo resonance. The intensity in each map is scaled independently for maximum contrast. Figure 1a shows the topography of single CuPc (top) and NiPc (bottom) on Ag(100), following evaporation in ultra-high vacuum (Methods). The molecules adsorb with the macrocycle plane parallel to the surface and rotated by±30° with respect to the [110] direction. The mistmatch between molecular and surface symmetry directions induces a chiral distortion of the molecular orbitals [11] . Negligible hybridization of the d x 2- y 2 orbital with the substrate hinders charge transfer towards either Cu or Ni atoms, preserving the spin of the central metal ions [12] . This is in contrast to molecules that include Mn, Fe, and Co ions, where empty d -orbitals projecting outside the molecular plane directly hybridize with the substrate, leading to either quenching [13] , [14] , [15] , [16] , [17] or Kondo screening [18] , [19] of the metal spin. Figure 1: Structure and electronic properties of paramagnetic CuPc and diamagnetic NiPc adsorbed on Ag(100). ( a ) STM image of single CuPc (top, I =72 pA, V b =−5 mV) and NiPc (bottom, I =100 pA, V b =−3 mV), image size 2.5 nm×2.5 nm. The diagram superposed to NiPc indicates the position of the metal (orange), C (grey), N (blue), and H (white) atoms. ( b ) d I /d V spectra of CuPc (top) and NiPc (bottom) around E F measured on benzene (blue dot) and ( c ) on Cu and Ni ions (red dot) (setpoint: I =2 nA/1.1 nA, V b =−100 mV for CuPc/NiPc). Labels denote Kondo resonances of different nature: zero-bias ( K ), triplet–singlet ( K ts ), and vibrational ( K v ). Black solid lines in c are fits to the data using the sum of Lorentzian (blue) and step functions (shaded). ( d ) d 2 I /d V 2 spectra of CuPc (top) and NiPc (bottom) measured on Cu and Ni ions. The dashed lines indicate the energy of the step excitations in c , which correspond to the amplitude of the Raman-active vibrational modes of gas-phase CuPc (bars) [21] . ( e ) Extended d I /d V spectra of CuPc on benzene and ( f ) Cu sites (setpoint: I =3 nA, V b =−2 V). ( g ) d I /d V maps of the molecular orbitals and inelastic vibrational signal shown in e and f together with the d 2 I /d V 2 map of the Kondo resonance. The intensity in each map is scaled independently for maximum contrast. Full size image Adsorption-induced ligand spin and delocalized Kondo effect Figure 1 illustrates the starting point of this work, namely the observation of a ligand spin induced by adsorption, which is delocalized over the peripheral atoms of both CuPc and NiPc. Differential conductance (d I /d V ) spectra acquired at 4.8 K on the outer benzene rings of the molecules reveal a strong zero-bias resonance ( Fig. 1b ), which reduces drastically towards the molecule centre ( Fig. 1c ). The scaling of the resonance amplitude and full width at half maximum ( Γ K ) indicates the presence of a screened magnetic moment [3] , [20] with Kondo temperature T K =27±2 K for CuPc and 29±2 K for NiPc ( Fig. 2 ). The spectra recorded over Cu and Ni ions, on the other hand, are dominated by sharp conductance steps at finite bias, symmetrically distributed around the Fermi level ( Fig. 1c ). As shown by the d 2 I /d V 2 curves in Figure 1d , the step energies correspond to the vibrational modes of CuPc and NiPc that involve a distortion of the metal–N bond [21] ( Supplementary Note 1 ), inelastically excited by electron tunnelling [22] . Our observations thus indicate that the screened spin is not localized on the metal ion, contrary to conclusions generally drawn from molecular junction experiments [1] , [2] , [3] and studies of metal–organic complexes at surfaces [16] , [18] , [19] , [23] , [24] , but induced by charge transfer into molecular ligand states [13] , [25] , [26] , [27] , [28] , independently of the spin of the pristine molecules. 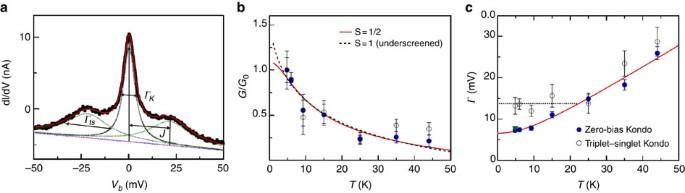Figure 2: Triplet–singlet excitations and temperature dependence of the CuPc Kondo resonance. (a) dI/dVspectrum measured at 4.8 K and fit of the zero-bias intensity and triplet–singlet side peaks (setpoint:I=2 nA,Vb=−100 mV). (b) Intensity (G) of the zero-bias and triplet–singlet conductance peaks as a function of temperature normalized by the conductance measured at 4.8 K (G0). The solid (dashed) line is a fit ofG/G0for theS=1/2 (underscreenedS=1) Kondo model obtained within the numerical renormalization group approach3, withTK=27 K. (c) Temperature dependence of the zero-bias and triplet–singlet resonance widthsΓK(filled symbols) andΓts(open symbols), respectively. The solid line is a fit ofΓKaccording to ref.20, resulting inTK=27 K. Figure 2: Triplet–singlet excitations and temperature dependence of the CuPc Kondo resonance. ( a ) d I /d V spectrum measured at 4.8 K and fit of the zero-bias intensity and triplet–singlet side peaks (setpoint: I =2 nA, V b =−100 mV). ( b ) Intensity ( G ) of the zero-bias and triplet–singlet conductance peaks as a function of temperature normalized by the conductance measured at 4.8 K ( G 0 ). The solid (dashed) line is a fit of G/G 0 for the S =1/2 (underscreened S =1) Kondo model obtained within the numerical renormalization group approach [3] , with T K =27 K. ( c ) Temperature dependence of the zero-bias and triplet–singlet resonance widths Γ K (filled symbols) and Γ ts (open symbols), respectively. The solid line is a fit of Γ K according to ref. 20 , resulting in T K =27 K. Full size image d I /d V measurements performed over a broader energy range offer further insight into the origin of the Kondo-screened magnetic moment. Figure 1e,f compare extended d I /d V spectra of CuPc recorded on Cu (red) and benzene (blue). The highest occupied (HOMO) and lowest unoccupied (LUMO) molecular orbitals of the gas-phase Pc macrocycle can be easily identified here. Both are extended π -orbitals with a 1 u and 2 e g symmetry, respectively, without significant mixing with d -states. The only orbital with d -metal character around the Fermi level, namely the b 1 g ( d x 2- y 2 ) state, cannot be directly observed because of its small overlap with the STM tip states. Charge transfer from the Ag substrate to the molecules results in the partial occupation of the gas-phase LUMO, which appears as a double-peak structure separated by 0.65 eV around the Fermi level ( E F ). This is characteristic of a partially filled orbital with Coulomb repulsion U separating the states with single- and double-electron occupancy. The Coulomb energy U=0.65 eV agrees with that expected for the π -orbitals of purely aromatic complexes [29] , [30] . Density functional theory (DFT) calculations support the identification of the molecular orbitals reported in Figure 1e–g ( Supplementary Note 2 ). 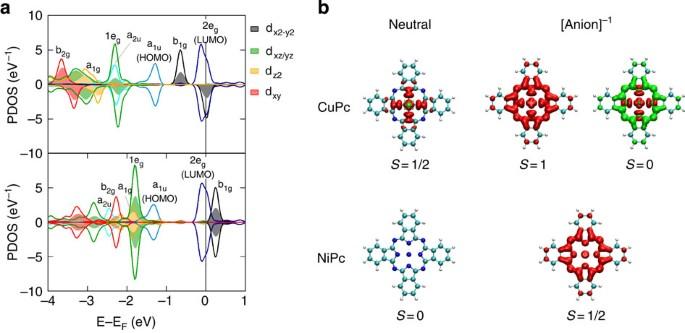Figure 3: Projected density of states (PDOS) and intramolecular exchange coupling. (a) PDOS of CuPc and NiPc on Ag(100) calculated by DFT. The projection onto the different molecular orbitals is given by solid lines; shaded areas indicate the metald-character of each state. (b) Spin density of neutral and anionic CuPc and NiPc species in the gas-phase. The sign of the spin is indicated in red/green. The density of states projected onto the different molecular orbitals of CuPc on Ag(100), shown in Figure 3a , reveals the HOMO lying at about −1.3 eV below E F and the Fermi level crossing of the LUMO. In agreement with the conclusions drawn from the experiment, we find that approximately one electron transfers from the substrate to the LUMO of both CuPc and NiPc species. We note that the double-peak LUMO structure observed in the d I /d V spectra cannot be reproduced by DFT because of the notorious underestimation of correlation effects in delocalized orbitals intrinsic to this method. On the other hand, the calculations show that the higher repulsion energy and the extremely low coupling of the d x 2- y 2 state to the substrate prevent substantial charge transfer to this orbital, leaving the spin of the Cu and Ni ions unperturbed. Figure 3: Projected density of states (PDOS) and intramolecular exchange coupling. ( a ) PDOS of CuPc and NiPc on Ag(100) calculated by DFT. The projection onto the different molecular orbitals is given by solid lines; shaded areas indicate the metal d -character of each state. ( b ) Spin density of neutral and anionic CuPc and NiPc species in the gas-phase. The sign of the spin is indicated in red/green. Full size image By comparing d I /d V maps at the energy of the HOMO, LUMO, and Kondo resonances, reported in Figure 1g , we can univocally assign the character of the ligand spin appearing in CuPc and NiPc as being due to the unpaired electron occupying the 2 e g LUMO state. This is demonstrated by the striking match of the symmetry and intensity of the LUMO and Kondo maps, as well as by the presence of the two 'Coulomb-blockade' peaks corresponding to the LUMO and LUMO+ U states around the zero-bias Kondo resonance. The ligand spin is thus delocalized around the molecule periphery, following the spatial distribution of the LUMO. We note that this orbital has also a small but finite weight at the molecule centre ( Fig. 3b ), which agrees with the low-intensity zero-bias Kondo resonance observed in Figure 1c . It is interesting to contrast our results with those of other molecules showing a delocalized Kondo resonance. Previous STM studies have shown that TCNQ molecules that are part of a mixed TTF–TCNQ layer also present a zero-bias Kondo peak due to charge transfer into a molecular orbital [29] . In such a case, however, charge transfer occurs from the TTF to the TCNQ molecules, following the well-known donor/acceptor character of these complexes established from bulk measurements. In our case, charge transfer and the corresponding ligand spin are induced at the single-molecule level through hybridization with the substrate. Measurements performed on CuPc adsorbed on Au(111), reported in Supplementary Note 3 , show that the interaction with the substrate is critical in this respect, as the LUMO remains above E F and we do not observe a Kondo effect for this surface. Another relevant point is that, within the error, T K does not present significant spatial variations, as expected for spin flip events involving a single-electron orbital. This is remarkably different from the adsorption-induced delocalization of the metal spin observed previously in Co porphyrin complexes on Cu(111), for which T K has been found to vary strongly over the porphyrin radius [13] , [17] . Moreover the total magnetic moment of the Co porphyrins does not change on deposition on Cu, whereas it increases by about 1 μ B for CuPc and NiPc on Ag. In such a case, because the LUMO is orthogonal to the metal d -orbitals, the Cu and Ni spins are not affected by adsorption and the extra spin occupies a purely ligand orbital. Intramolecular resolution of metal–ligand spin coupling The presence of both metal and ligand spins in the same molecule opens up the possibility to investigate inter-orbital spin coupling with intramolecular resolution, a central result of this work. We find that, in CuPc, the π -spin couples to the d -spin forming singlet (S=0) and triplet (S=1) states. The fingerprints of this interaction are the two side peaks observed at E Kts =±21 meV (±1 meV) in the d I/ d V spectrum of CuPc, which are absent in NiPc ( Figs 1b and 2a ). In Kondo systems, such side peaks are assigned to cotunnelling events that involve coherent Kondo spin-flips and inelastic excitations [31] . 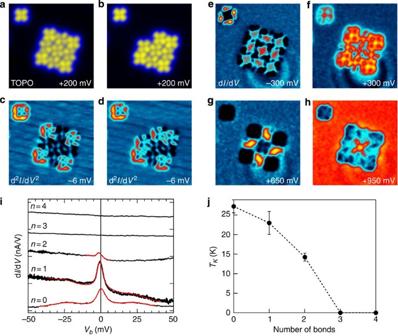Figure 4: Influence of intermolecular interactions. (a) and (b) STM image of a 3x3 cluster of CuPc before and after removing a corner molecule by manipulation with the tip. (c) and (d) Kondo resonances simultaneously mapped with the images inaandb. Note that the Kondo resonance can be observed only for molecules with a number of lateral bonds smaller than three. (e–h) Molecular orbital conductance maps show the correlation between molecular coordination, energy shift of the LUMO, and disappearance of the Kondo effect. (i) Conductance spectra acquired at 4.8 K at the benzene ring of molecules with different number of side-to-side neighbours and in different configurations. (j) Evolution of the Kondo temperature with the number of intermolecular bonds. Unlike quantum dots, where the reduced orbital level-spacing may favour the coupling of Kondo and electronic excitations [32] , [33] , the origin of such side peaks in small aromatic molecules is restrained to vibrational [5] , [27] , [29] or magnetic [34] , [35] , [36] excitations, as schematized in Figure 4a . We observe several side peaks in the d I /d V spectra of CuPc and NiPc. At the Cu and Ni sites ( Fig. 1c ), these peaks coincide with the inelastic conductance steps due to vibrational excitations ( Fig. 1d ) and can therefore be assigned to vibrational Kondo events [26] . The coupling mechanism is analogous to that discussed for other aromatic molecules [27] , [29] . Note that the same peaks are observed for CuPc and NiPc independently of their spin moment, as the vibrational spectrum of the two molecules is identical. The side peaks observed at the benzene sites ( Fig. 1b ), on the other hand, are a unique feature of CuPc and can only be assigned to intramolecular magnetic excitations. This conclusion agrees with the fact that CuPc contains two spins, whereas NiPc has only one, as shown previously. The energy of the CuPc side peaks thus provides a direct measurement of the intramolecular exchange coupling J = E Kts between π and d spins. The observation of an intense Kondo peak at zero bias, rather than a valley, indicates that the molecule ground state is magnetic, namely a triplet state where the metal and ligand spin are aligned parallel to each other. Figure 4: Influence of intermolecular interactions. ( a ) and ( b ) STM image of a 3x3 cluster of CuPc before and after removing a corner molecule by manipulation with the tip. ( c ) and ( d ) Kondo resonances simultaneously mapped with the images in a and b . Note that the Kondo resonance can be observed only for molecules with a number of lateral bonds smaller than three. ( e–h ) Molecular orbital conductance maps show the correlation between molecular coordination, energy shift of the LUMO, and disappearance of the Kondo effect. ( i ) Conductance spectra acquired at 4.8 K at the benzene ring of molecules with different number of side-to-side neighbours and in different configurations. ( j ) Evolution of the Kondo temperature with the number of intermolecular bonds. Full size image This picture is supported also by DFT calculations of the magnetic structure of gas-phase [CuPc] −1 , where the anion configuration is used to model the main effect of the substrate, that is, the transfer of approximately one electron into the CuPc orbitals. In the gas-phase, the energies of S =0 and S =1 configurations can be conveniently computed by fixing the total spin of the molecule. The calculations show that, in addition to the b 1 g spin of the free molecule, the anion has an extra spin localized over the LUMO, which couples parallel to the first one ( Fig. 3b ). From the energy difference between the triplet ground state and the (antiparallel) singlet state, a value of J =36 meV can be extracted for the exchange coupling constant. This energy is larger than the triplet–singlet excitation energy found for CuPc on Ag(100), which can be easily explained by the reduced correlation expected for molecular orbitals hybridized with metal states. Note that similar calculations for [NiPc] −1 yield a spin-polarized LUMO with S =1/2 and no other spin degree of freedom, forbidding inelastic magnetic excitations in the absence of a magnetic field. Underscreened Kondo effect of CuPc Although the spin moments of CuPc and NiPc are different, the two molecules exhibit similar Kondo temperatures. This is related to the fact that in CuPc only the ligand spin couples to conduction electrons of the substrate, providing a single screening channel. The effective decoupling of the d x 2- y 2 orbital, confined in the molecular plane, leads to an underscreened Kondo state, where the total spin S =1 reduces to S =1/2 (refs 3 , 35 , 37 ). This is part of a two-stage process, where the presence of a strongly coupled and a weakly coupled screening channel implies the existence of two different Kondo energy scales [35] , [37] . In the temperature range accessible to our experiment, only the LUMO screening channel is effective, which explains why the measured Kondo temperature is similar for CuPc and NiPc. Indeed, fitting the intensity of the CuPc Kondo resonance using analytic expressions derived from renormalization group theory for the S =1/2 and the underscreened S =1 Kondo effect [3] yields results that are consistent with this interpretation, as shown in Figure 2c and further discussed in Supplementary Note 4 . Our measurements indicate that the residual spin of CuPc is not screened until temperatures much lower than 4.8 K. Influence of molecule–molecule interactions A point of interest in characterizing the coupling of metal–organic complexes to a metal is the influence of intermolecular interactions. Previous studies have shown that the Kondo temperature of metal–organic complexes can be manipulated by locally modifying the ligand field acting on the transition-metal ions [3] , [38] or by screening the surface electron density around molecular adsorbates by other molecules [39] . Here we show that the presence of the ligand spin, hence the total spin of CuPc and NiPc, depends on the number of lateral bonds and can be artificially manipulated by assembling molecular clusters of different size and shape ( Supplementary Note 5 ). Figure 4 reports the topography and spectroscopic maps of a 3×3 square cluster of CuPc molecules. A single molecule close to the upper left corner serves as a control reference. Images and spectra show that the Kondo resonance survives only in the molecules at the four corners, which have N =2 lateral neighbours. The relationship between T K and N is further proven by removing one of the corner molecules ( Fig. 4b ) as well as by fabricating chain- and cross-shaped clusters, which reveal the quench of the Kondo effect for N ≥3 ( Fig. 4c, d ). The explanation of this effect lies in the strong dependence of substrate–molecule charge transfer on N , and the abrupt disappearance of the ligand spin in molecules having N ≥3 neighbours. Figure 4e–h shows that, although no clear LUMO profile can be detected at V =−0.3 V, the corner molecules still display the characteristic intensity distribution around the aromatic ligand in correspondence of the LUMO+ U orbital ( V =+0.3 V). Molecules with N =3 display a new intense resonance peaking at +650 mV, and for N =4, the energy of this peak is shifted to +950 mV. These spectral features are narrower and more intense compared with those observed for N <3, indicating the gradual decoupling of the molecules from the substrate. Accordingly, such resonances are assigned to the upshift of the LUMO, which is accompanied by a redistribution of the electron density specific to each bonding configuration. As the LUMO completely crosses E F , the ligand spin disappears, closing the spin-dependent transport channels of the molecules. Spatial distribution of spin and vibrational excitations Taking advantage of the spatial and energy resolution afforded by STM, the different nonequilibrium conductance resonances found in CuPc can be mapped along an axis that runs from the molecule centre towards its periphery. 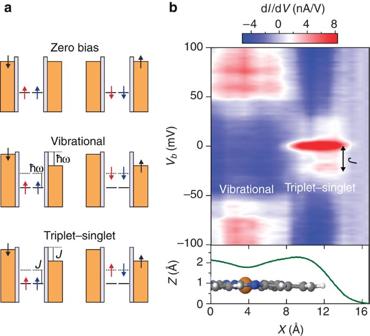Figure 5: Site-specific conductance of spin and vibrational co-tunnelling processes. (a) Schematic of the cotunnelling mechanisms giving rise to zero-bias, vibrational, and triplet–singlet Kondo resonances. (b) Intramolecular conductance: dI/dVspectra measured along a line crossing the Cu ion and a benzene ring (horizontal axis) as a function ofVb(vertical axis) (stabilization setpoint:I=1 nA,Vb=−100 mV). Red-coloured regions illustrate the different localization of the Kondo excitation channels. Note the abrupt transition from vibrational to triplet–singlet excitations at ~4 Å away from the Cu site. The results, shown in Figure 5 , demonstrate that the vibrational and triplet–singlet inelastic channels occupy mutually exclusive regions both in energy and space, with the former localized on the central part of the molecule and the latter on the external ring structure. The localization of the vibrational coupling around the ion site is related to the distortion of Cu–N bonds in all excited modes [40] ( Supplementary Note 1 ). On the other hand, the intensity of the triplet–singlet excitations is proportional to the local spin/charge density as well as to the probability to tunnel to spin-polarized orbitals, the latter being much higher for the LUMO. Thus, as the STM tip has the role of a mobile electrode, our measurements show that the appearance of nonlinear resonances in the I / V curves of metal–organic complexes is related in a nontrivial way to the contact geometry with the metal leads and to the vibronic and magnetic degrees of freedom within the molecules. Figure 5: Site-specific conductance of spin and vibrational co-tunnelling processes. ( a ) Schematic of the cotunnelling mechanisms giving rise to zero-bias, vibrational, and triplet–singlet Kondo resonances. ( b ) Intramolecular conductance: d I /d V spectra measured along a line crossing the Cu ion and a benzene ring (horizontal axis) as a function of V b (vertical axis) (stabilization setpoint: I =1 nA, V b =−100 mV). Red-coloured regions illustrate the different localization of the Kondo excitation channels. Note the abrupt transition from vibrational to triplet–singlet excitations at ~4 Å away from the Cu site. Full size image Relaxation and universal scaling of nonequilibrium Kondo excitations The coexistence of different nonequilibrium Kondo processes related to vibrational excitations at energies E Kv1 , E Kv6 and a triplet–singlet transition at E Kts opens multiple relaxation channels for the CuPc ligand spin. The interplay of different many-body excitations represents a formidable challenge for the theoretical description of the spin and current dynamics in small quantum objects coupled to external charge reservoirs, which has been difficult to address experimentally [41] . Here CuPc provides the opportunity to compare spin relaxation via vibrational and magnetic cotunnelling events in the same molecule. To do so, we deconvoluted the inelastic tunnelling conductance of purely vibrational origin from the vibrational Kondo finite-bias intensity by fitting the d I /d V spectra of CuPc and NiPc using the sum of six-step functions and Lorentzian curves on each side of E F ( Fig. 1c ; Supplementary Note 1 ). The triplet–singlet excitation features were modelled by two Lorentzian peaks as shown in Figure 2a . The full width at half maximum of the triplet–singlet peaks ( Γ ts ) and vibrational resonances ( Γ v ) is inversely related to the decoherence time of the co-tunnelling processes schematized in Figure 5a . At temperature T ≥ T K , both Γ ts and Γ v are dominated by thermal broadening, similar to Γ K . Deeper into the Kondo regime, however, we observe that Γ ts deviates from Γ K , saturating at 14 meV ( Fig. 2c ). This demonstrates that the intrinsic timescales of triplet–singlet and zero-bias Kondo spin flips are different. Such finding led us to investigate the scaling properties of the conductance as a function of T K and V b . Current theoretical models assert that nonequilibrium Kondo physics is completely universal and determined by a single energy scale corresponding to T K (ref. 42 ). Universality, however, applies uniquely to the elastic Kondo resonance, hence there is no physical reason for Kondo processes that involve different type of inelastic excitations to obey the same decoherence rate as a function of energy. A major hurdle to prove this point lies in the need of comparing data relative to triplet–singlet [3] , [35] and vibrational excitations [2] , [29] for different systems, especially in experiments where the electrode–molecule coupling and Kondo temperature greatly differ from each other. Such a comparison can be carried out by renormalizing both Γ and V b by the relevant Kondo energy scales for each system, that is, by plotting Γ/Γ K as a function of V b / k B T K , in analogy with the theory of dc-biased quantum dots [42] . 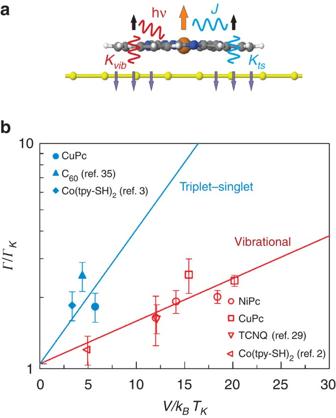Figure 6: Spin versus vibrational relaxation channels. (a) Diagram showing the spin distribution and couplings of CuPc induced by adsorption on Ag. (b) Normalized widthΓ/ΓKof the inelastic Kondo resonances as a function ofVb/kBTK. Data for CuPc and NiPc are compared with that for other molecules for which either spin or vibrational Kondo excitations have been separately reported. Triplet–singlet (cyan) and vibrational (red)Kondo excitations separate into two groups. Exponential fits (solid lines) evidence the different contribution of each process to the decoherence rate. Figure 6 shows the renormalized Γ ts and Γ v values of CuPc and NiPc, obtained in this way. We find that Γ v follows the exponential trend with V b expected for the relaxation of nonequilibrium Kondo processes that are dominated by electron-hole pair excitations [34] , [43] . However, Γ ts of CuPc lies outside this trend, showing a larger normalized decoherence rate compared with vibrational excitations. Data from experiments separately reporting singlet-triplet [3] , [35] and vibrational [2] , [29] Kondo features in systems with T K differing by as much as two orders of magnitude also support this conclusion. Figure 6 shows that finite-bias resonances related to vibrational excitations fit a single exponential curve (red line) with a decay rate that is a factor 3 smaller compared with inelastic spin excitations (cyan line), reflecting the different decay channels present in each case. We conclude that the coherence of nonequilibrium Kondo cotunnelling events is universal only when restricted to the subspace of a given observable. Indeed, the faster decoherence, observed for the triplet–singlet channel, can be related to the higher coupling of the electron bath to spin excitations as compared with phonon excitations [44] , and might apply to other types of nonequilibrium Kondo phenomena, including those involving Cooper pairs or photon adsorption [45] , [46] . Figure 6: Spin versus vibrational relaxation channels. ( a ) Diagram showing the spin distribution and couplings of CuPc induced by adsorption on Ag. ( b ) Normalized width Γ/Γ K of the inelastic Kondo resonances as a function of V b / k B T K . Data for CuPc and NiPc are compared with that for other molecules for which either spin or vibrational Kondo excitations have been separately reported. Triplet–singlet (cyan) and vibrational (red)Kondo excitations separate into two groups. Exponential fits (solid lines) evidence the different contribution of each process to the decoherence rate. Full size image Bias and temperature are the parameters that define the transport properties of ideal molecular conductors. The interaction with metal contacts brings about substantial changes to the molecular conductance. As demonstrated here, such changes are not only due to the symmetry-allowed matching of substrate and molecular orbitals, but also by deep modifications of the molecular magnetic structure. An apparently simple molecule/metal system thus turns out to be very complex entity in terms of magnetism and electron transport. Our results illustrate how orbital- and site-specific interactions determine the spin multiplicity of the molecular junction and the type of inelastic excitations that dominate spin dynamics at low energies. We also find that the probability of exciting different vibrational and magnetic excitations varies with sub-angstrom scale inside a single molecule, showing how the molecular conductance depends abruptly on the precise position of the molecule–metal contact. The competition between Kondo, vibrational and magnetic excitations determines the decoherence rate of the molecular spin. Finally, we showed that interactions between molecules have a role analogous to that of an electrostatic gate, inducing strong shifts of the electronic levels with respect to E F in molecular clusters of controlled size and shape. These understandings are essential for the design of molecular spintronic devices. Sample preparation CuPc and NiPc molecules were evaporated in ultra-high vacuum on single crystal Ag(100). The substrate was prepared by repeated sputter–anneal cycles using Ar+ ions at an energy of 700 eV and annealing to 800 K. The molecules were deposited at a rate of ~0.05 monolayers per min with the sample kept at room temperature, after degassing the 99% pure powder material (Sigma Aldrich) to 500 K for 24 h. The base pressure during evaporation was below 5×10 −10 mbar. STM measurements were carried out at the base temperature of 4.8 K, and up to 35 K for the temperature-dependence study of the Kondo resonance. The adsorption and self-assembly of CuPc on Ag(100) have been previously studied in detail [11] . NiPc molecules behave as CuPc. The molecules adsorb parallel to the substrate plane with two different azimuthal orientations corresponding to a rotation of the molecular axis of +30° and −30° (±2°) relative to the [011] surface lattice direction, with the Cu and Ni ions occupying Ag hollow sites in both cases. STM spectroscopy d I /d V measurements were carried out with the lock-in technique, using bias voltage modulation with frequency between 2 and 3 kHz and rms amplitude of 1 mV for the short-range spectra focusing on low-energy features, and 3 mV for the larger range spectra used to probe the molecular orbitals far away from E F . Possible instrumental contributions to the linewidth were checked by decreasing the voltage modulation down to 250 μV without noting any difference. Background spectra acquired on the bare Ag surface, using the same feedback parameters as for the on-molecule spectra, have been subtracted to all the d I /d V curves reported in this paper in order to remove electronic features due to the substrate and tip ( Supplementary Methods ). The frequency used in the second derivative measurements varied between 745 Hz and 1.5 kHz, and a voltage modulation of 3 mV was used in this case. Ab-initio calculations We performed electronic structure calculations of individual CuPc and NiPc molecules adsorbed on Ag(100) to complement the information obtained from STM spectroscopy. We used the VASP implementation of DFT in the projector-augmented plane–wave scheme and the local density approximation. The calculated slabs include five Ag atomic layers intercalated by seven vacuum layers in the vertical direction, and a 7×7 lateral supercell. The positions of all atoms in the molecule and the first three Ag layers were relaxed vertically and laterally until forces were smaller than 0.01 eV Å −1 . How to cite this article: Mugarza, A. et al . Spin coupling and relaxation inside molecule-metal contacts. Nat. Commun. 2:490 doi: 10.1038/ncomms1497 (2011).